Rational design of all organic polymer dielectrics To date, trial and error strategies guided by intuition have dominated the identification of materials suitable for a specific application. We are entering a data-rich, modelling-driven era where such Edisonian approaches are gradually being replaced by rational strategies, which couple predictions from advanced computational screening with targeted experimental synthesis and validation. Here, consistent with this emerging paradigm, we propose a strategy of hierarchical modelling with successive downselection stages to accelerate the identification of polymer dielectrics that have the potential to surpass ‘standard’ materials for a given application. Successful synthesis and testing of some of the most promising identified polymers and the measured attractive dielectric properties (which are in quantitative agreement with predictions) strongly supports the proposed approach to material selection. Polymeric dielectric materials are pervasive in modern electronics and electrical systems. They have found applications in the areas of capacitive energy storage [1] , [2] , [3] , [4] , [5] , [6] , transistors [7] , [8] , [9] , photovoltaic devices [10] , [11] , [12] and electrical insulation [13] , [14] . The selection and design of a polymer depends on the requirements specific to the application, which, in the case of dielectric applications, can be stated in terms of a subset of the following properties: dielectric constant, band gap, dielectric breakdown field, dielectric loss, morphology, glass transition temperature, mechanical strength, cost and so on. Although the property requirements can be specified with reasonable precision, trial and error strategies (aided by chemical intuition or serendipity) have dominated the identification or discovery of suitable candidates that meet such requirements. While successful, these strategies suffer from the fact that they are not generalizable, and discoveries (and, equally importantly, the lack of such prospects) cannot be rigorously assessed. The community is thus gradually migrating towards systematic computation-driven materials (down) selection paradigms [15] , [16] . Consider, for instance, the case of polymers for capacitive energy storage applications. The on-going electrification of land [17] , [18] and sea [19] transportation, as well as other military and civilian systems [19] , [20] has increased the demand for high energy density capacitors. The choice of polymers (over ceramics) in capacitive energy storage applications is motivated by the need for ‘graceful failure’ of the dielectric at high fields. Metallized polymers offer the only scalable capacitor technology that meets this need. The energy stored in a capacitor is proportional to the dielectric constant and the square of the electric field. Thus, materials of interest should display a high dielectric constant and high electrical breakdown field. In addition, low dielectric loss and resistance to high field degradation of the polymer itself are important requirements as well. The present state-of-the-art in high energy density metalized film capacitors employ biaxially oriented polypropylene (BOPP), which has a small area (~1 cm 2 ) breakdown field of about 750 MV m −1 and a dielectric constant of about 2.2. Various attempts to replace BOPP have been based on poly(vinyledene fluoride) (PVDF) and its copolymers [1] , [21] , [22] , polymer nanocomposites [23] , [24] , [25] and so on. All such potential replacements have suffered from either high loss (PVDF and its copolymers) or low breakdown field (nanofilled polymers). A strategy is needed to identify promising new polymers. In this contribution, we present a rational design strategy of hierarchical modelling with successive downselection stages to efficiently screen and identify advanced polymer dielectrics for capacitive energy storage applications. Specifically, quantum mechanics-based combinatorial searches of chemical space are used to identify polymer repeat units that could lead to desirable dielectric properties, followed by configurational space searches using evolutionary and classical molecular dynamics schemes to determine the three-dimensional (3D) arrangement of polymers (and their properties) built from the desirable repeat units. Successful synthesis and testing of some of the most promising identified polymers and the measured attractive dielectric properties supports the proposed approach to material selection. Overview In essence, we show that a systematic combinatorial search of the polymer chemical and configurational spaces can lead to new polymers with attractive combinations of properties. By chemical space, we refer to the various building blocks (‘monomers’) in the polymer, while configurational space encompasses the connectivity sequences possible with these building blocks, the manner in which the resulting chains pack together, and the larger scale morphology. In a first line of screening attempted in this work, we identify attractive polymers based on their dielectric constant and band gap values, both of which can be computed with reasonable accuracy using quantum mechanical computations. As noted earlier, dielectrics for high energy density capacitor applications need to satisfy additional requirements, including low dielectric loss and high dielectric breakdown strength (thus making the presently adopted screening criteria necessary but not sufficient conditions). Since the current state-of-the-art does not allow us to determine these attributes quantitatively in a high-throughput framework, we use the band gap as a proxy. Recent work suggests that large values of the intrinsic breakdown strength of a variety of insulators are correlated with large band gap values [26] , [27] . Besides, the band gap and dielectric constant, in and of themselves, are important properties in a variety of applications. Our step-by-step computational search strategy to arrive at promising polymeric dielectrics is depicted schematically in Fig. 1 . This strategy includes the following successive (and to some extent, iterative) steps: (1) Combinatorial chemical space exploration using 1D polymer chains with four independent blocks per repeat unit; (2) Promising repeat unit (that is, sequence of blocks) identification based on band gap and dielectric constant estimates; (3) 3D structure/morphology predictions of polymers composed of the downselected repeat units; (4) Property predictions of the 3D systems; and (5) Synthesis of the identified polymers, followed by testing and validation. Steps 3–5 are time-intensive. Hence, candidates identified in Step 2, which are amenable to synthesis, are favored in Steps 3–5. 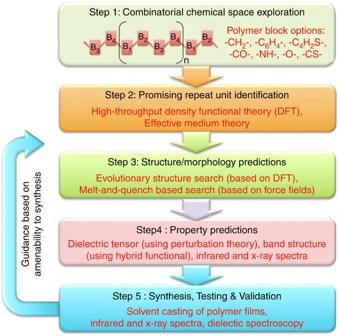Figure 1: A schematic illustration of our rational polymer dielectric design strategy. The strategy involves five consecutive steps: (1) Combinatorial chemical space exploration, using 1D polymer chains containing four independent blocks with periodic boundary conditions along the chain axis, (2) Promising repeat unit identification, by screening based on band gap and dielectric constant, (3) 3D structure/morphology predictions of polymers composed of the downselected repeat units, (4) Property predictions of the 3D systems. Finally, (5) Synthesis testing and validation. Application of this strategy to the design of organic polymeric dielectrics for high energy density applications has identified several polymers, some of which (especially those with prior evidence of synthesis success) are listed in Table 1 . The top three members of Table 1 have also been synthesized by us, and appear attractive based on the measured dielectric properties. In what follows, we describe the details of our search strategy in a step-by-step manner. Figure 1: A schematic illustration of our rational polymer dielectric design strategy. The strategy involves five consecutive steps: (1) Combinatorial chemical space exploration, using 1D polymer chains containing four independent blocks with periodic boundary conditions along the chain axis, (2) Promising repeat unit identification, by screening based on band gap and dielectric constant, (3) 3D structure/morphology predictions of polymers composed of the downselected repeat units, (4) Property predictions of the 3D systems. Finally, (5) Synthesis testing and validation. Full size image Table 1 Promising polymer repeat units identified at Step 2 of the screening process. Full size table Combinatorial chemical space exploration The first level of screening involves the 1D catenation of repeat units into a polymer chain. In the present search, repeat units were constructed using four building blocks in the repeat unit with each block drawn from the following pool of possibilities: -CH 2 -, -C 6 H 4 -, -C 4 H 2 S-, -NH-, -CO-, -O-, -CS-, as depicted in Fig. 1 . These blocks were chosen because they are common in polymer backbones, including polyethylene, polyesters, polyamides, polyethers and polyureas. After the elimination of obviously unstable combinations of these building blocks (such as systems containing contiguous -CO- or -O- blocks) and accounting for translational and inversion symmetry, we were left with 267 unique repeat units (c.f. Supplementary Table 1 ). Density functional theory (DFT) computations were performed to determine the optimal 1D structure of each of these systems, followed by the estimation of the electronic and ionic contributions to the dielectric constant by a combination of density functional perturbation theory (DFPT) and effective medium theory [28] , [29] . The latter approach is critical as it allows us to estimate the dielectric constant of a macroscopic polymer based just on its 1D structure, as explained previously [28] , [29] . 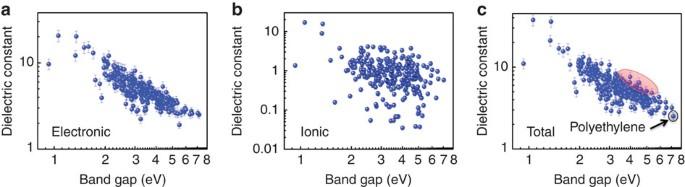Figure 2: The dielectric constant versus band gap relationship of 1D polymers. Computed (a) electronic, (b) ionic and (c) total dielectric constant (along the polymer chain axis) as a function of the band gap. The associated errors in the dielectric constant computed using density functional perturbation theory for single chains, and subsequently estimated using effective medium theory for a bulk environment are also shown. The highlighted region corresponds to the most ‘promising repeat units’ composed of at least one of -NH-, -CO- and -O-, and at least one of -C6H4- and –C6H2S- blocks. Band gap was computed using the HSE06 electronic exchange-correlation functional. Promising repeat unit identification Figure 2 portrays the relationship between the dielectric constant (electronic, ionic and total) and the band gap for the 267 polymers, including the prototypical system, polyethylene (when all four blocks are set to -CH 2 -), which has the largest band gap and the smallest dielectric constant of all systems studied. As can be seen from Fig. 2a , the upper bound of the electronic part of the dielectric constant versus the band gap data displays a near perfect inverse dependence. This imposes a theoretical limit on the achievable electronic part of the dielectric constant, a limit that can be understood by regarding this property as related to a sum over electronic transitions from occupied to unoccupied states [30] . On the other hand, the ionic part of the dielectric constant, which is determined by the infrared (IR)-active zone centre phonon modes (that is, the modes that display a time-varying dipole moment) [31] , [32] , is not correlated with the band gap, as seen from Fig. 2b . The ionic dielectric constant can thus be exploited to increase the total dielectric constant without compromising the band gap. Figure 2: The dielectric constant versus band gap relationship of 1D polymers. Computed ( a ) electronic, ( b ) ionic and ( c ) total dielectric constant (along the polymer chain axis) as a function of the band gap. The associated errors in the dielectric constant computed using density functional perturbation theory for single chains, and subsequently estimated using effective medium theory for a bulk environment are also shown. The highlighted region corresponds to the most ‘promising repeat units’ composed of at least one of -NH-, -CO- and -O-, and at least one of -C 6 H 4 - and –C 6 H 2 S- blocks. Band gap was computed using the HSE06 electronic exchange-correlation functional. Full size image Figure 2c , which shows the variation of the total dielectric constant with the band gap, is a ‘map’ of the achievable combination of these properties within the chemical space explored. Capacitive energy storage and some electronics applications, for example, gate insulations, could draw from the large dielectric constant and moderate band gap region of this plot. As illustrated in Fig. 2c , downselection, starting from the set of 267 polymers with four-block repeat units, proceeded by considering the polymers with total dielectric constant >~4 eV and band gap >~3 eV. Polymers that survive this initial screening step are predominantly composed of at least one of the polar units, namely -NH-, -CO- and -O-, and at least one of the aromatic rings, namely -C 6 H 4 - and -C 6 H 2 S-. -NH-, -CO- and -O- tend to enhance the ionic part of the dielectric constant, while the aromatic groups boost the electronic part. A selected assortment of these promising polymers (especially those with prior evidence of synthesis success) are listed in Table 1 in decreasing order of total dielectric constant. Interestingly, none of these specific polymers have been considered in the past for dielectric applications, although a few other polymers in the general classes listed in Table 1 (for example, polythiourea [6] ) have been shown to hold promise for dielectric applications. Structure/morphology prediction We now consider only the top three downselected cases of Table 1 , namely, [-NH-CO-NH-C 6 H 4 -] n , [-CO-NH-CO-C 6 H 4 -] n and [-NH-CS-NH-C 6 H 4 -] n . The 3D structure of these three polymers was determined using two complementary approaches: (1) a version of the Universal Structure Predictor: Evolutionary Xtallography (USPEX) method [33] , [34] , [35] , [36] , [37] specially modified to handle repeat units rather than atoms as the building blocks, and (2) a classical molecular dynamics based melt-and-quench approach. The former used DFT energetics (here used with 4 repeat units per unit cell) and hence provide ground state (0 K) results, while the latter used a newly generated force field and hence could treat much larger systems containing thousands of repeat units per unit cell at nonzero temperatures. Both the modified USPEX [36] , [37] and the melt-and-quench schemes lead to several low energy configurations, which were equivalent within the expected uncertainties of the force-field and DFT energy predictions. This is reassuring as it indicates that the ground state structures predicted by DFT are expected to be stable at higher temperatures as well. 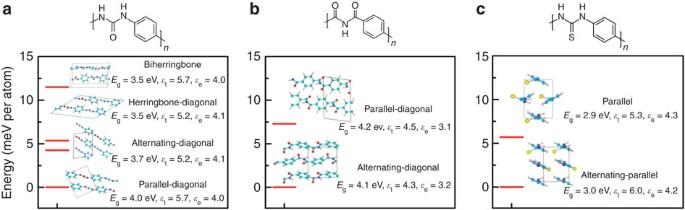Figure 3: Predicted properties and structures of the identified promising polymers. The repeat units of the three identified polymers are (a) [-NH-CO-NH-C6H4-] (b) [-CO-NH-CO-C6H4-] and (c) [-NH-CS-NH-C6H4-]. The crystal structures of [-NH-CO-NH-C6H4-] are predicted by evolutionary structure search (using DFT) and melt-and-quench (using force-field (FF)) schemes, while in other two polymers only evolutionary structure search (using DFT) method has been used. The zero of the energy scale corresponds to the most stable structures. For each predicted structure, the calculated values of the band gap (Eg), total (εt) and electronic (εe) part of dielectric constants are also listed. Figure 3 shows the energetic ordering of a few low energy structures for each of the three polymers considered at this stage. Figure 3: Predicted properties and structures of the identified promising polymers. The repeat units of the three identified polymers are ( a ) [-NH-CO-NH-C 6 H 4 -] ( b ) [-CO-NH-CO-C 6 H 4 -] and ( c ) [-NH-CS-NH-C 6 H 4 -]. The crystal structures of [-NH-CO-NH-C 6 H 4 -] are predicted by evolutionary structure search (using DFT) and melt-and-quench (using force-field (FF)) schemes, while in other two polymers only evolutionary structure search (using DFT) method has been used. The zero of the energy scale corresponds to the most stable structures. For each predicted structure, the calculated values of the band gap ( E g ), total ( ε t ) and electronic ( ε e ) part of dielectric constants are also listed. Full size image Simulated X-ray diffraction (XRD) and infrared (IR) spectra based on the predicted low energy structures for all three polymers are presented in Figs 4 , 5 , 6 , and discussed and compared with measurements below. 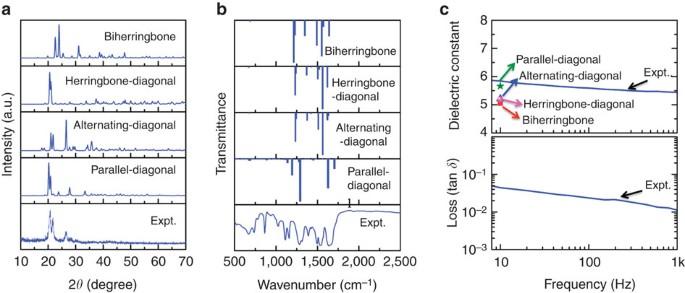Figure 4: Experimental and predicted data for the polymer with repeat unit [-NH-CO-NH-C6H4-]. (a) X-ray diffraction data (b) IR spectra, and (c) dielectric spectra (top panel) and loss factor (bottom panel). Expt, experimental. Figure 4: Experimental and predicted data for the polymer with repeat unit [-NH-CO-NH-C 6 H 4 -]. ( a ) X-ray diffraction data ( b ) IR spectra, and ( c ) dielectric spectra (top panel) and loss factor (bottom panel). Expt, experimental. 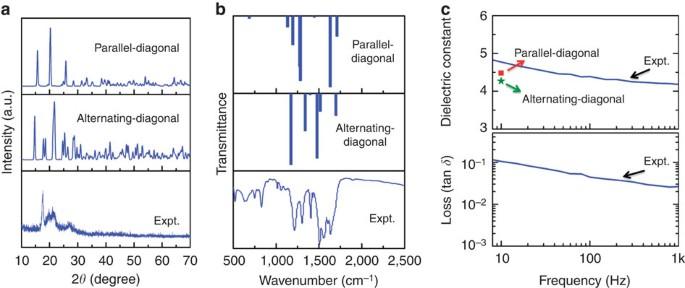Figure 5: Experimental and predicted data for the polymer with repeat unit [-CO-NH-CO-C6H4-]. (a) X-ray diffraction data (b) IR spectra, and (c) dielectric spectra (top panel) and loss factor (bottom panel). Expt, experimental. Full size image Figure 5: Experimental and predicted data for the polymer with repeat unit [-CO-NH-CO-C 6 H 4 -]. ( a ) X-ray diffraction data ( b ) IR spectra, and ( c ) dielectric spectra (top panel) and loss factor (bottom panel). Expt, experimental. 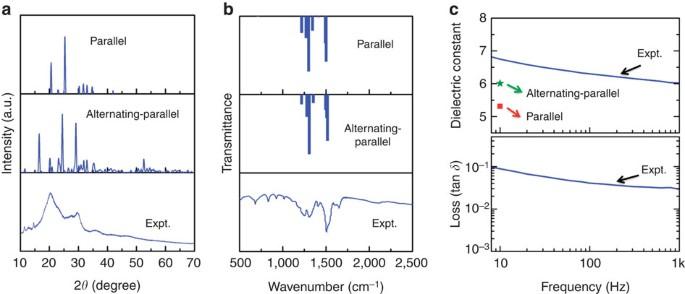Figure 6: Experimental and predicted data for the polymer with repeat unit [-NH-CS-NH-C6H4-]. (a) X-ray diffraction data (b) IR spectra, and (c) dielectric spectra (top panel) and loss factor (bottom panel). Expt, experimental. Full size image Figure 6: Experimental and predicted data for the polymer with repeat unit [-NH-CS-NH-C 6 H 4 -]. ( a ) X-ray diffraction data ( b ) IR spectra, and ( c ) dielectric spectra (top panel) and loss factor (bottom panel). Expt, experimental. Full size image Property predictions The computed band gap values of all the identified low energy structures are listed in Fig. 3 . As can be seen, except in the case of [-NH-CS-NH-C 6 H 4 -] n , the band gap ( E g ) values are over 3.5 eV for all identified structures. Computed electronic band structure and density of states are shown in Supplementary Information (c.f. Supplementary Figure 1 ). The dielectric constants were determined using DFPT, with results for the orientational average ranging from 4 to 6, double that of polyethylene or polypropylene. The electronic part of the dielectric constant for all polymers ranges from 3 to 4, placing these with polymers that display the highest known refractive indices [38] . Assuming that the predicted ground state structures remain stable at elevated temperatures close to room temperatures (a reasonable assumption based on the discussion above), the predicted band gaps and dielectric constants are expected to be valid at those elevated temperatures as well. In situations when amorphous polymeric phases are expected in reality (aided by competing energetics or favourable kinetics), some deviations in the dielectric constant with respect to those predicted here is to be expected. Nevertheless, as dielectric behaviour is generally dominated by local chemistry and bonding, the deviations are expected to be small (see discussion below pertaining to the [-CO-NH-CO-C 6 H 4 -] n and [-NH-CS-NH-C 6 H 4 -] n polymers). The predicted values of the total ( ε t ) and electronic ( ε e ) parts of dielectric constants for all three polymers considered are listed in Fig. 3 . As can be seen, the fidelity of the predictions of Step 2 persist at Step 4 of our process (insofar as the band gap and dielectric constant values are concerned). Validation through synthesis and testing Synthesis of the [-NH-CO-NH-C 6 H 4 -] n , [-CO-NH-CO-C 6 H 4 -] n and [-NH-CS-NH-C 6 H 4 -] n polymers proceeded via adaptation of previous efforts [39] . Measurements were performed on pressed pellets of the synthesized polymers. The measured band gap values of the three polymers are 3.9 eV, 4.0 eV and 3.1 eV, respectively, in good agreement with the predictions listed in Fig. 3 . Considering [-NH-CO-NH-C 6 H 4 -] n first ( Fig. 4a ), a characteristic double peak in the XRD spectra at 2θ≈20° can be seen for all the predicted structures except the ‘biherringbone’ case, in line with the measurements, with the agreement being best for the ‘parallel-diagonal’ case. The correspondence between the measured IR spectrum ( Fig. 4b ) and that of the four predicted structures is uniformly good. This is not surprising as the IR peaks are dominated by intra-chain ‘bonded’ interactions. Such interactions are roughly the same for all four predicted structures, which differ largely only in the manner in which the individual chains are packed. Based on these findings, we conclude that the [-NH-CO-NH-C 6 H 4 -] n polymer is dominated by regions of ‘parallel-diagonal’ structure, although smaller portions of the other three structures cannot be ruled out at or close to room temperatures. Figure 4c portrays the dielectric spectrum for the synthesized [-NH-CO-NH-C 6 H 4 -] n polyurea system. Across a wide frequency range, the dielectric constant is in the 5.4–5.8 range, and the dielectric loss at 1 kHz is in the range of 1%, an acceptable value for some applications. Figure 4c also shows the computed average (over all directions) total dielectric constant values for all four predicted [-NH-CO-NH-C 6 H 4 -] n crystal structures. Once again, the agreement between measurement and predictions is excellent. The predicted XRD spectra of the [-CO-NH-CO-C 6 H 4 -] n , and [-NH-CS-NH-C 6 H 4 -] n polymers ( Figs 5a and 6a ) do not match well with the measured spectra, which display broad peaks. This indicates that the synthesized and cast [-CO-NH-CO-C 6 H 4 -] n and [-NH-CS-NH-C 6 H 4 -] n polymers are in semicrystalline or amorphous form. On the other hand, the measured and calculated IR spectra ( Figs 5b and 6b ) are in good agreement for both [-CO-NH-CO-C 6 H 4 -] n and [-NH-CS-NH-C 6 H 4 -] n for the same reasons identified above in the discussion of the [-NH-CO-NH-C 6 H 4 -] n polymer. The measured dielectric constant of [-CO-NH-CO-C 6 H 4 -] n is in the range of 4.2–4.8 and that of [-NH-CS-NH-C 6 H 4 -] n is in the 5.7–6.7 range, both in good agreement with predictions (shown in Figs 5c and 6c , and in Fig. 3 ), despite the fact that the predictions are made for the crystalline varieties of these polymers. Both polymers display dielectric loss larger than that of the [-NH-CO-NH-C 6 H 4 -] n . We have outlined a rational procedure for systematically exploring polymer chemical spaces and identifying potentially useful dielectrics based on the dielectric constant and band gap as initial screening criteria. This procedure is computationally driven (with ample guidance from chemical intuition and synthesis considerations) and uses a combination of quantum mechanical calculations, force-field simulations and structure and property prediction schemes in a hierarchical manner. A class of organic polymers involving seven distinct building blocks was screened using this approach and several promising polymers were identified. A common feature of these downselected polymers is the occurrence of at least one of the polar units, -NH-, -CO- and -O-, and at least one of the aromatic rings, -C 6 H 4 - and -C 6 H 2 S-. Three of the most promising cases were synthesized and tested. The favourable agreement between the measured and predicted (structural, electronic and dielectric) properties of all three polymers, and the low dielectric loss of one of these (namely, [-NH-CO-NH-C 6 H 4 -] n ) provides validation and hope for such a rational computationally driven approach for materials discovery. Indeed, processable variants of the polymers identified here are presently being further evaluated. While the present development is certainly a significant advance over empiricism, consistent with the emerging paradigm of computation-driven materials (down)selection [15] , [16] , it is only an initial attempt that should be extended by including other critical properties in the screening process. Such properties include dielectric loss, dielectric breakdown strength, mechanical behaviour, glass transition temperature and charge carrier mobility. The current state-of-the-art limits our ability to predict these properties rapidly and with high fidelity. It is hoped that recent advances in data-driven and first-principles methodologies will allow us overcome these limitations with time [16] , [40] . While the present effort has focussed primarily on high energy density capacitor dielectrics, polymers for other applications (for example, organic semiconductors or organic photovoltaics) can be identified in a systematic manner using an extended version of the present strategy by considering other relevant screening criteria and many types of blocks. First-principles computations The quantum mechanical computations were performed using DFT as implemented in the Vienna ab initio software package [41] , [42] . The generalized gradient approximation functional, parametrized by Perdew, Burke and Ernzerhof (PBE) [43] to treat the electronic exchange-correlation interaction, the projector augmented wave [44] potentials and plane-wave basis functions up to a kinetic energy cutoff of 500 eV, were employed. The supercells were relaxed using a conjugate gradient algorithm until the forces on all atoms were <0.02 eV Å −1 . As the PBE functional is known to underestimate band gaps of insulators, the Heyd−Scuseria−Ernzerhof HSE06 functional [45] was used to obtain corrected band gap values for all systems considered. The 1D systems considered in Step 1 were composed of all-trans infinitely long isolated chains containing four independent building units in a supercell geometry (with periodic boundary conditions along the axial direction). In a combinatorial and exhaustive manner, each block in the polymer backbone was allowed to be one of the following units: -CH 2 -, -NH-, -C(=O)-, -C 6 H 4 - (benzene), -C 4 H 2 S- (thiophene), -C(=S)- or -O-, which are commonly seen in polymer backbones [29] , [46] , [47] . The scheme results in 267 symmetry unique cases. A Monkhorst–Pack k -point mesh of 1 × 1 × k (with kc >50) was used to produce converged results for a supercell of length c (Å) along the chain direction (that is, the z direction). The stress component along the z direction was required to be <1.0 × 10 −2 GPa. The dielectric permittivity of the isolated polymer chains placed in a large supercell was first computed within the DFPT [48] , [49] formalism, which includes contributions from the polymer as well as from the surrounding vacuum region of the supercell. Next, treating the supercell as a vacuum-polymer composite, effective medium theory [50] was used to estimate the dielectric constant of just the polymer chains using methods described recently [28] , [29] . In the case of polymer crystals (discussed below), van der Waals interactions were taken into account using the vdW-TS functional [51] . Phonon dispersion curves were calculated using the supercell approach with the finite displacement method as implemented in the PHONOPY code [52] , while FullProf suite [53] was used to simulate the XRD patterns. Structure prediction using evolutionary algorithm A specifically designed constrained evolutionary algorithm [36] , [37] , embodied in the USPEX code [33] , [34] , [35] , [37] was used to predict polymeric crystal structures starting from the single polymeric chains discussed above (using first-principles quantum mechanical computations for the total ground state energy of the crystals). This newly developed method uses a specification of well-defined molecular repeat units rather than individual atoms as the starting point [36] . The diversity of the population of structures is enhanced by using space-group symmetry combined with random cell parameters, and random positions and orientations of the molecular units [36] , [37] . During the evolutionary optimization, structures with different sequence and packing of these repeat units are generated and relaxed. We performed multiple runs of evolutionary search with two and four repeat units. The total energies were obtained with the PBE exchange-correlation functionals using the dispersion correction prescribed by the vdW-TS approach [51] . In all cases considered here, the energetic orderings are invariant with respect to the choice of different exchange-correlation functionals. Structure prediction using the melt-and-quench scheme The simulations were performed using the LAMMPS molecular dynamics package [54] and the OPLS-2005 force field [55] . The polymer [-NH-CO-NH-C 6 H 4 -] n requires a torsion potential for N-C-N-CA (where CA is an aromatic carbon) which is not present in the force field. This potential was calculated using the molecule CO-(NH-C 6 H 4 ) 2 via fitting to the difference in energy, between using the force field and using Hartree–Fock 6-31G*, minimized under constraint of the two torsions of this type in a series of calculations to sweep out the full range of motion. To make the torsion potential fit all configurations satisfactorily, it was necessary to modify the atomic partial charges. These were set to match Mulliken charges scaled down by a factor of 1.86, and the charges of H and CA bonded to N were adjusted to ensure a good fit. Two kinds of simulations were performed, which differed in whether the polymers were terminated with an end group within the periodic cell or whether they were covalently bonded to the other end of the polymer via the periodic wrapping. The first set consisted of 18mer chains terminating in phenyl rings. A single chain was quenched into a straight conformation corresponding to the minimization of all bonds, angles and torsions. The single chain was replicated in a 6 × 6 rectangular array. The system was heated at 1 K ps −1 , and the structure was observed to change between 800 and 860 K. The 860 K configuration was selected for cooling at various rates. At the cooling rate of −10 K ps −1 , a ‘parallel’ crystal was produced with a ‘herringbone’ defect, but cooling at −1 ps −1 produced a perfect ‘parallel’ crystal. After further study, this melt-and-quench process was repeated starting with a perfect ‘parallel-diagonal’ crystal. During heating at 1 K ps −1 , this crystal underwent two transitions between 710 and 810 K before showing signs of melting at 850 K. The 820 K configuration cooled at either −1 or −0.1 K ps −1 yielded a ‘biherringbone’ crystal. The second set of simulations consisted of a 4 × 4 array of 4mer chains connected to themselves through the periodic boundary, making them effectively infinite. Owing to the periodic restriction, nematic order remains at very high temperatures (1,000 K). Crystals were obtained by cooling from this high-temperature state. The initial configuration of the crystals before heating is thus immaterial. Usually, the ‘herringbone’ configuration was obtained, in both fast (−10 K ps −1 ) and slow quenches (−0.05 K ps −1 ), but two cases resulted in ‘biherringbone’ configurations (−10 K ps −1 , −0.2 K ps −1 ). ‘Parallel’ crystals were never obtained after cooling if the system had been heated >900 K. Synthesis and characterization details For the synthesis of the first two polymers, namely, [-NH-CO-NH-C 6 H 4 -] and [-CO-NH-CO-C 6 H 4 -], a flame-dried, argon-flushed 125 ml round bottom flask equipped with a reflux condenser, gas inlet, magnetic stirbarand 50-ml dry dimethylsulphoxide were used. In the polyurea case [-NH-CO-NH-C 6 H 4 -], equimolar amounts of p- phenylene diisocyanate and p- phenylenediamine were used, while for the polyimide [-CO-NH-CO-C 6 H 4 -], equimolar amounts of terephthalamide and terephthaloyl chloride were used (35 mmol). The mixtures were heated at 350 K for 8 h under pre-purified argon, after which they were poured into dry tetrahydrofuran. The white solid precipitates were filtered and washed copiously in fresh tetrahydrofuran, followed by drying in vacuo . The yields for the polyurea and polyimide were nearly quantitative. The following synthesis route was adopted for the [-NH-CS-NH-C 6 H 4 -] polymer. To a dry 100 ml three-neck flask, 0.9614, g (5 mmol) of p- phenylene diisothiocyanate and 10 ml dry dimethylsulfoxide were added under nitrogen with stirring, followed by the addition of 0.5407, g (10 mmol) of p- phenylenediamine. The reaction was carried out at room temperature. After 6 h, a white powder crashed out of the solution. The mixture was poured into 150 ml of methanol, filtered and washed with methanol several times, and dried in vacuo . A white solid was obtained at 89% yield (1.337 g). XRD patterns were obtained on a Bruker D5005 X-ray diffractometer equipped with a 2.2 kW copper X-ray tube. The dielectric spectra were obtained on an IMASS time domain dielectric spectrometer. Measurements were taken by sandwiching a pressed pellet of material between silicone rubber guarded electrodes. Pellets were prepared in a hydraulic press with a 1 inch circular pellet mould. IR spectra were obtained on a Nicolet Magna-IR 560 spectrometer using KBr pellets, and the bandgaps were determined using optical data obtained on a Varian Cary 5000 UV/Visible spectrometer. How to cite this article: Sharma, V. et al. Rational design of all organic polymer dielectrics. Nat. Commun. 5:4845 doi: 10.1038/ncomms5845 (2014).